Electrically driven nanobeam laser The realization of lasers as small as possible has been one of the long-standing goals of the laser physics and quantum optics communities. Among multitudes of recent small cavities, the one-dimensional nanobeam cavity has been actively investigated as one of the most attractive candidates for effective photon confinement thanks to its simple geometry. However, the current injection into the ultra-small nano-resonator without critically degrading the quality factor remains still unanswered. Here we report an electrically driven, one-dimensional, photonic-well, single-mode, room-temperature nanobeam laser whose footprint approaches the smallest possible value. The small physical volume of ~4.6 × 0.61 × 0.28 μm 3 (~8.2( λ n −1 ) 3 ) was realized through the introduction of a Gaussian-like photonic well made of only 11 air holes. In addition, a low threshold current of ~5 μA was observed from a three-cell nanobeam cavity at room temperature. The simple one-dimensional waveguide nature of the nanobeam enables straightforward integration with other photonic applications such as photonic integrated circuits and quantum information devices. In recent years, high-quality ( Q ) factor, small mode volume ( V ), ultrasmall lasers/resonators have been actively investigated for both fundamental and practical applications [1] . For example, various two-dimensional (2D) photonic crystal lasers have been demonstrated through optical and electrical pumping [2] , [3] , [4] , [5] , [6] , [7] , [8] , [9] , [10] , [11] , [12] , [13] . The physical volume of these small lasers, however, is limited by the area of the photonic crystal lattice surrounding the cavity of interest, and the physical footprints are typically >10 μm 3 (refs 2 , 3 , 10 , 11 ). Sub-wavelength scale plasmonic lasers have also been demonstrated [14] , [15] , [16] , [17] , [18] , [19] , [20] . However, in these metallic structures, the unavoidable ohmic losses had critical roles and lasing action was observed mostly at low temperature through optical and electrical pumping. Therefore, a low-loss, small-volume, metal-free cavity has been sought after for more efficient and acceptable photon confinement. Recently, one-dimensional (1D) nanobeam cavities have been widely investigated as one of the more attractive candidates for a small high- Q resonator [21] , [22] , [23] , [24] , [25] , [26] , [27] , [28] , [29] . Thanks to its inherent 1D nature, a 1D photonic bandgap can always be formed regardless of the material choice. When a nanobeam is constructed from a high-index semiconductor material, a high- Q resonator can be easily realized with a small number of air holes. Moreover, with the proper choice of resonant mode that overlaps less with the air holes, one can minimize the non-radiative surface recombination effect. The simple and robust 1D waveguide structure of the nanobeam is expected to enable straightforward integration with other photonic applications such as photonic integrated circuits [27] , optomechanical devices [28] and quantum information devices [29] . However, the problem of current injection into this small footprint nanobeam for laser diode operation without critically degrading the Q factor of the resonator still remains to be solved. In this article, we demonstrate an electrically driven, photonic-well, metal-free, 1D nanobeam laser whose physical footprint approaches the smallest possible. Design and fabrication of the nanobeam lasers As the dimension of a resonator approaches the order of the wavelength of light or less, it becomes increasingly more difficult to confine photons efficiently in the small space. Among the many resonant modes available in various 1D nanobeam cavity structures with large Q / V values, we focus our attention to the ones that are compatible with current injection. It is known that 1D or 2D photonic wells can be constructed by modulating the photonic band structures of the surrounding region [12] , [13] , [24] . In order to confine photons more efficiently in the smaller volume, we employ the photonic well by grading the size of the central air holes, as shown in Fig. 1a . Between the two available bands, those modes originating from the air band are chosen for two practical reasons. The first is that, in the nanobeam structure, the only available location for the electrode is in the region between the air holes. Those air band modes with intensity nodes at the position of the InP electrodes are expected to experience smaller optical losses. Second, the smaller central air holes are critical for the formation of the central under-lying posts by preferential wet chemical etching which is diffusion-limited. 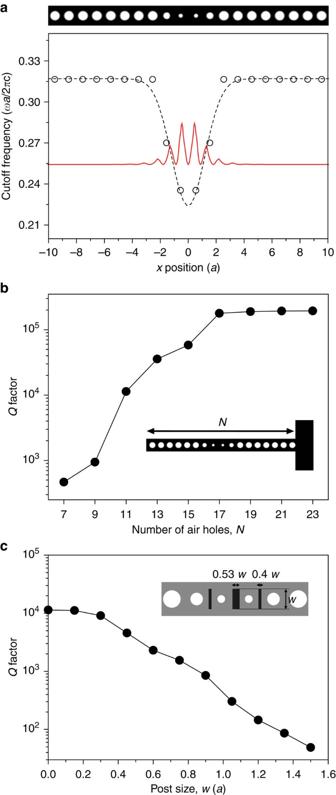Figure 1:Photonic well 1D nanobeam resonator. (a) Plot of the cutoff frequency of guided modes as a function of thexposition of the nanobeam (black dotted line). A resonant mode is found in the photonic well at a normalized frequency of 0.254 (red line). In the computation, the radii of air holes are 0.15aat the centre, 0.25ain the next-nearest holes, and 0.35ain all other holes, whereais the lattice constant. The distance between the two central holes is shifted by 1.10a. The width and thickness of the nanobeam are 1.5aand 0.7a, respectively. (b)Qfactors of free-standing photonic well resonators as a function of the total number of air holes,N. We add one more air hole to the right side of the nanobeam cavity to compensate for the optical loss at the nanobeam-dielectric slab boundary (inset). (c)Qfactors of the photonic well resonator withN=11 as a function of the sizewof the underlying post. The areas of the central post and side post are 0.53w×wand 0.4w×w, respectively, wherewchanges from 0 to 1.5a, which is the nanobeam width. Figure 1: Photonic well 1D nanobeam resonator . ( a ) Plot of the cutoff frequency of guided modes as a function of the x position of the nanobeam (black dotted line). A resonant mode is found in the photonic well at a normalized frequency of 0.254 (red line). In the computation, the radii of air holes are 0.15 a at the centre, 0.25 a in the next-nearest holes, and 0.35 a in all other holes, where a is the lattice constant. The distance between the two central holes is shifted by 1.10 a . The width and thickness of the nanobeam are 1.5 a and 0.7 a , respectively. ( b ) Q factors of free-standing photonic well resonators as a function of the total number of air holes, N . We add one more air hole to the right side of the nanobeam cavity to compensate for the optical loss at the nanobeam-dielectric slab boundary (inset). ( c ) Q factors of the photonic well resonator with N =11 as a function of the size w of the underlying post. The areas of the central post and side post are 0.53 w × w and 0.4 w × w , respectively, where w changes from 0 to 1.5 a , which is the nanobeam width. Full size image Q factors of various nanobeam cavities are calculated and compared to identify the optimum size and the total number ( N ) of air holes ( Fig. 1b ). Typically the Q factor increases rapidly for N >9 and is saturated for N ≥17. It is found that Q factors >1,000 can be obtained with N ≥11 ( Fig. 1b ). Thus, the photonic cavity of N =11 was chosen for further analyses. However, the introduction of the central posts is expected to degrade the Q factor of the resonator. For practical reasons, the effect of the central InP posts should also be studied in detail. As expected, optical losses increase with the size ( w ) of the post, which is defined in the inset of Fig. 1c . It is encouraging to find that reasonable Q factors >1,000 are obtainable with a reasonable post size of w <0.75 a ( Fig. 1c ), where a is the lattice constant of the nanobeam. The final structure of choice consists of only 11 graded air holes and a post size of half of the nanobeam width which falls within our fabrication capability. It is significant that such strong light confinement occurs in an ultra-small cavity with a physical volume of ~4.6 × 0.61 × 0.28 μm 3 . It is worth pointing out that this length of the 11 air holes agrees reasonably with the room-temperature carrier diffusion length [30] . Based on the above cavity design shown in Fig. 1 , an electrically driven nanobeam laser structure is fabricated as shown in the schematic diagram of Fig. 2a . A submicron-sized semiconductor post and a metal electrode are used as p - and n -contacts, respectively. Electrons and holes injected into the n - i - p InGaAsP slab containing three quantum wells are recombined in the proximity of the InP post which falls within the hole diffusion length ( Fig. 2b ). The fabrication procedure is as follows (see also Supplementary Fig. S1 ). First, an AuGe n -contact electrode with a thickness of 100 nm and area of 5 × 30 μm 2 is deposited onto the n - i - p InGaAsP substrate. The electrode is annealed at 250 °C for 10 min in a vacuum chamber for ohmic contact. Then trench patterns are defined on the slab around the electrode using electron-beam lithography followed by chemically assisted ion-beam etching. Next, the InP sacrificial layer underneath the slab, except for the region where a photonic crystal cavity is formed, is removed selectively by wet etching using HCl solution. This etched region is filled with dielectric material, photoresist, which acts as both a current block and a mechanical support layer after the hardening process. The nanobeam structure connected to the n -contact electrode is subsequently fabricated using additional electron-beam lithography and dry etching processes. Finally, single or three-legged submicron-sized central InP posts are formed underneath the nanobeam cavity by diffusion-limited, anisotropic, low-temperature wet etching based on diluted HCl solution (HCl:H 2 O=3:1) at 10 °C. 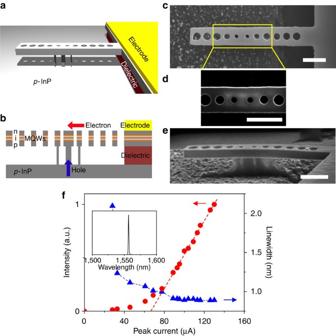Figure 2:Electrically driven photonic well nanobeam laser. (a) Schematic diagram of an electrically driven nanobeam laser. (b) Schematic diagram showing the injection of electrons and holes into the nanobeam cavity. Ann-i-pslab structure including three InGaAsP QWs is used. (c) Top-view SEM image of a fabricated nanobeam structure. Only 11 air holes are used to achieve lasing. (d) Magnified top-view SEM image of (c). One can see the post underneath the slab at a high SEM voltage. (e) Tilted-view SEM image of the nanobeam structure. The scale bars inc–eare all 1 μm. (f) Measured output power (red circles) and linewidth (blue triangles) as a function of injected peak current. The lasing threshold is ~65 μA. The inset shows an above-threshold lasing spectrum. Single-mode lasing is observed at a wavelength of 1,556 nm. Figure 2: Electrically driven photonic well nanobeam laser . ( a ) Schematic diagram of an electrically driven nanobeam laser. ( b ) Schematic diagram showing the injection of electrons and holes into the nanobeam cavity. An n - i - p slab structure including three InGaAsP QWs is used. ( c ) Top-view SEM image of a fabricated nanobeam structure. Only 11 air holes are used to achieve lasing. ( d ) Magnified top-view SEM image of ( c ). One can see the post underneath the slab at a high SEM voltage. ( e ) Tilted-view SEM image of the nanobeam structure. The scale bars in c – e are all 1 μm. ( f ) Measured output power (red circles) and linewidth (blue triangles) as a function of injected peak current. The lasing threshold is ~65 μA. The inset shows an above-threshold lasing spectrum. Single-mode lasing is observed at a wavelength of 1,556 nm. Full size image To control the size and position of the InP post reliably, we take advantage of the anisotropic and slow etching characteristics of InP crystal at low temperature [2] , [3] , [31] . As the sacrificial InP layer tends to be under-etched preferentially along the <100> crystallographic directions by HCl-based etchants, the nanobeam length is aligned along the <100> direction ( Supplementary Fig. S2 ). The three sub-micron-size posts are formed underneath the regions between the smaller central air holes owing to the diffusion-limited nature of the wet etching process. Figure 2c–e show top- and tilted-view scanning electron microscope (SEM) images of a typical fabricated sample. This post structure, which is properly aligned and reproducible, enables selective current injection into the nanobeam cavity with minimal tolerable additional optical scattering losses of the cavity mode ( Supplementary Fig. S3 ). Measurement of lasing characteristics The fabricated nanobeam laser structure is electrically pumped with 10-ns current pulses at a period of 1 μs at room temperature. Injected electrons and holes recombine near the central posts, emitting light at wavelengths near 1,550 nm. The electroluminescence (EL) is collected by a × 50 long-working-distance microscope objective (numerical aperture of 0.42) and imaged onto either a spectrometer or an infrared camera. To confirm lasing, the output power and the spectral linewidth are measured as functions of the peak current ( Fig. 2f ). With increasing pump current, the spectral width of the EL decreases continuously and becomes saturated at a value of 0.9 nm once it reaches the lasing threshold (blue triangles in Fig. 2f ). Single-mode lasing is observed at a wavelength of 1,556 nm (inset of Fig. 2f ). The transverse electric-like output is linearly polarized along the direction perpendicular to the length of the nanobeam. The measured lasing threshold current is ~65 μA (red circles in Fig. 2f ). For a better understanding of the experimental observation, we performed the three-dimensional (3D) contour finite-difference time-domain (FDTD) analysis using the digitized SEM image data of the fabricated nanobeam structure shown in Fig. 2c . One can notice that the measured image of the lasing mode of interest ( Fig. 3a ) agrees closely with the vertical component of time-averaged Poynting vector convolved with the resolution of the objective ( Fig. 3b ). Through the contour FDTD analyses, we find that the slightly shifted single-intensity lobe is attributable to the asymmetrically fabricated structure. Efficient light confinement in the nanobeam is also confirmed as shown in Fig. 3c . The Q factor and mode volume are calculated to be ~650 and 0.35( λ n −1 ) [3] , respectively, which includes fabrication imperfections faithfully. 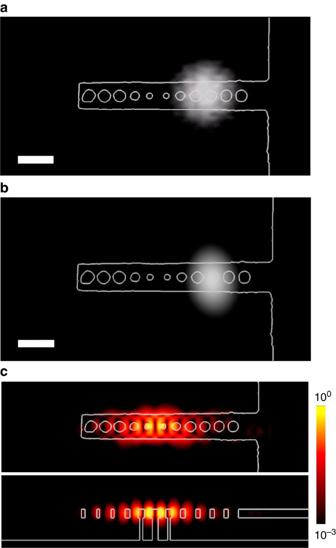Figure 3:Lasing mode profile of the photonic well nanobeam laser. (a) Lasing mode profile captured by an infrared camera. (b) Calculated vertical component of time-averaged Poynting vector distribution at a position 3.6 μm above the slab, which represents those propagating photons that have escaped from the bound mode shown in (c). The scale bars in (a,b) are 1 μm. (c) Top and side views of the calculated mode profile of log |E|2. The SEM image ofFig. 2cis used for this simulation. The resonant wavelength of the mode is 1,588 nm. Figure 3: Lasing mode profile of the photonic well nanobeam laser . ( a ) Lasing mode profile captured by an infrared camera. ( b ) Calculated vertical component of time-averaged Poynting vector distribution at a position 3.6 μm above the slab, which represents those propagating photons that have escaped from the bound mode shown in ( c ). The scale bars in ( a , b ) are 1 μm. ( c ) Top and side views of the calculated mode profile of log | E | 2 . The SEM image of Fig. 2c is used for this simulation. The resonant wavelength of the mode is 1,588 nm. Full size image Three-cell nanobeam lasers For comparison purposes, larger nanobeam cavity structures were also investigated. For example, a tapered three-cell nanobeam cavity was formed by filling in three central air holes and slightly reducing the size of two air holes near the cavity ( Fig. 4a ). The somewhat larger central post is shown in the tilted-view SEM image ( Fig. 4b ). The radii of the regular and reduced air holes are 0.25 a and 0.15 a , respectively, and the nanobeam width is 1.5 a , where a is the lattice constant of 370 nm. In fact, this larger structure is optimized for a lower threshold and more air holes than used in the previous case. When the three-cell nanobeam structure is electrically pumped under pumping conditions identical to those in the former case, single-mode lasing is observed at a wavelength of 1,578 nm (inset of Fig. 4c ). In addition, the output power and linewidth of the mode are measured as a function of the injected current ( Fig. 4c ). A low room-temperature lasing threshold current of ~5 μA is observed. The linewidth changes abruptly near the threshold, and decreases to the resolution limit of the spectrometer, ~0.5 nm, above the threshold. The lower threshold of the three-cell cavity in comparison to that of the former cavity is ascribed to the higher Q factor, ~1,500, and the smaller surface recombination losses ( Supplementary Fig. S4 ). The peak voltage is measured as a function of the injected peak current, to elucidate the electrical properties of the nanobeam laser ( Supplementary Fig. S5 ). 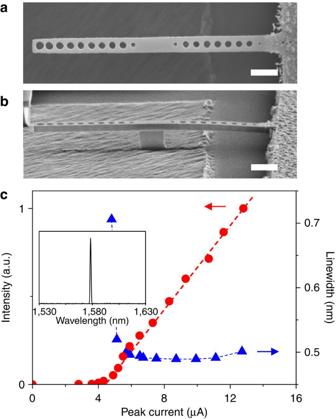Figure 4:Low-threshold tapered three-cell nanobeam laser. (a,b) Top- and tilted-view SEM images of a fabricated three-cell nanobeam structure. The scale bars are 1 μm. (c) Measured output power (red circles) and linewidth (blue triangles) as a function of injected peak current. The lasing threshold is ~5 μA. The lasing wavelength is 1,578 nm (inset). The average output power measured at the spectrometer is 24 pW at 12.8 μA. The corresponding wall-plug efficiency is estimated to be 0.5%, when an objective lens of numerical aperture of 0.42 was used. Figure 4: Low-threshold tapered three-cell nanobeam laser . ( a , b ) Top- and tilted-view SEM images of a fabricated three-cell nanobeam structure. The scale bars are 1 μm. ( c ) Measured output power (red circles) and linewidth (blue triangles) as a function of injected peak current. The lasing threshold is ~5 μA. The lasing wavelength is 1,578 nm (inset). The average output power measured at the spectrometer is 24 pW at 12.8 μA. The corresponding wall-plug efficiency is estimated to be 0.5%, when an objective lens of numerical aperture of 0.42 was used. Full size image The lasing characteristics of the single-cell and two-cell optically pumped nanobeam lasers are summarized in the Supplementary Information ( Supplementary Fig. S6 ). We also examined the lasing threshold of the nanobeam laser using simple rate equation analysis including non-radiative surface recombination [32] ( Supplementary Fig. S7 ) and found that the threshold of the 1D three-cell nanobeam laser is significantly lower than that of a 2D photonic crystal laser with the same structural and material parameters as the 1D nanobeam. As smaller active area requires lower current injection to make it transparent, the nanobeam laser whose active area is an order of magnitude smaller than 2D photonic crystal lasers can have lower threshold current [2] , [3] . In addition, low non-radiative surface recombination in the nanobeam laser can contribute to reducing threshold. In summary, we demonstrated an electrically driven, photonic well 1D nanobeam laser with a footprint approaching the smallest possible value achievable from metal-free cavities. In addition, we claim the lowest electrical threshold of ~5 μA at room temperature from the three-cell nanobeam cavity. The proposed 1D nanobeam lasers can be integrated with each other ( Supplementary Fig. S8 ) or can be combined with other nanophotonic devices such as waveguides and detectors thanks to its simple geometry. We believe that this nanolaser could be an essential element as an acceptable photon source for compact photonic integrated circuits and/or quantum information sciences. Wafer structure Nanobeam structures were fabricated using (280-nm thick n - i - p InGaAsP slab)/(1-μm thick p -InP sacrificial layer)/(100-nm thick p -InGaAs etch stop layer)/( p -InP substrate) wafer structure. Three InGaAsP multi-quantum wells were embedded in the middle of the slab. In addition, in the n - i - p InGaAsP slab, the doping densities of the top Si-doped n -layer and the bottom Zn-doped p -layer were ~2.0 × 10 19 and ~2.2 × 10 18 cm −3 , respectively. The absorption coefficients of the n - and p -layers at 1,550 nm are ~62 and ~50 cm −1 , respectively [33] . EL and PL measurements The fabricated nanobeam lasers were pumped electrically or optically with 10 ns current pulses at a period of 1 μs at room temperature, with no intentional cooling. For optical pumping, a 980 nm laser diode was used as a pumping source. The light emitted from the nanobeam structures was collected by a × 50 long-working-distance objective lens with a numerical aperture 0.42, focused onto either a spectrometer or an infrared camera. FDTD calculations We use home-built 3D FDTD simulations in Figs 1 and 3 , and Supplementary Fig. S4 . The refractive index of the InGaAsP slab and InP post was set to be 3.4. A uniaxial perfectly matched layer was used for the absorbing boundaries. In Fig. 3 and Supplementary Fig. S4 , mode profiles are calculated using the structures taken directly from the SEM images of the fabricated nanobeams, and thus all imperfections in fabrication are included. How to cite this article: Jeong, K.-Y. et al. Electrically driven nanobeam laser. Nat. Commun. 4:2822 doi: 10.1038/ncomms3822 (2013).